Contact ofcis-Golgi with ER exit sites executes cargo capture and delivery from the ER Protein transport from the endoplasmic reticulum (ER) to the Golgi apparatus is mediated by coat complex II (COPII) vesicles. It has been believed that COPII vesicles containing cargo are released from the ER exit sites (ERES) into the cytosol and then reach and fuse with the first post-ER compartment, cis- Golgi or ER-to-Golgi intermediate compartment (ERGIC). However, it still remains elusive how cargo loading to vesicles, vesicle budding, tethering and fusion are coordinated in vivo . Here we show, using extremely high speed and high resolution confocal microscopy, that the cis -Golgi in the budding yeast Saccharomyces cerevisiae approaches and contacts the ERES. The COPII coat cage then collapses and the cis -Golgi captures cargo. The cis- Golgi, thus loaded with cargo, then leaves the ERES. We propose that this ‘hug-and-kiss’ behaviour of cis- Golgi ensures efficient and targeted cargo transport from the ERES to cis- Golgi. The basic mechanism of endoplasmic reticulum (ER)-Golgi traffic is conserved from yeast to higher animals and plants, but the number, size and dynamics of the ER exit sites (ERES) and Golgi vary across cell types and species [1] , [2] . Most of the first post-ER compartments are located in the vicinity of the ERES. In C. elegans [3] , plant cells [4] and also the yeast P. pastoris [5] , which have separate stacks of flattened cisternae in the cytoplasm, the cis face of Golgi stacks show stable association with the ERES. In mammalian cells, Golgi stacks are clustered and connected with each other, forming a large Golgi ribbon in the perinuclear region. However, ER-to-Golgi intermediate compartment (ERGIC) is found near the ERES, which locate not only in the perinuclear region but also on the ER spreading throughout the cell [6] . The yeast S. cerevisiae presents a unique example. Specifically, individual Golgi cisternae, cis , medial and trans , do not stack but scatter in the cytoplasm [7] , [8] . Our previous findings indicated that, among Golgi cisternae moving around in the cytoplasm, cis- Golgi has higher probability of staying in the vicinity of the ERES than trans- Golgi [8] . To understand the significance of this behaviour of yeast Golgi, we employed an extremely high speed and high resolution microscopy technique, super-resolution confocal live imaging microscopy (SCLIM), that we recently developed [4] , [8] , [9] . ER-to- cis- Golgi and ER-to-ERGIC traffic has been believed to operate in a way that ER-derived COPII vesicles are once released into the cytosol and then get tethered to and fuse with neighbouring cis- Golgi or ERGIC [10] , [11] . Our observations, including visualization of cargo, challenge this model. In S. cerevisiae, cis -Golgi approaches and contacts the ERES and, concomitantly with the collapse of COPII coats, captures cargo and then leaves the ERES. cis- Golgi shows approach-and-contact actions toward the ERES We first conducted simultaneous dual-colour time-lapse observation of the ERES and cis- and trans- Golgi cisternae. ERES is defined as the place where COPII coat assembles, and thus Sec13, a COPII outer coat protein, was tagged with green fluorescent protein (GFP) and used as an ERES marker. Sed5, a SNARE (soluble N-ethylmaleimide-sensitive factor attachment protein receptor) molecule residing mainly in the cis- Golgi [12] , [13] , and Sec7, a guanine-nucleotide exchange factor for Arf GTPases primarily localizing in the trans- Golgi [14] , [15] , were fused with monomeric red fluorescent protein (mRFP) [16] and used as cis- and trans -Golgi markers, respectively. Sec13-GFP showed a typical organized feature of S. cerevisiae ERES with relatively stable localization [8] , [17] , whereas Golgi cisternae were much more mobile [7] , [8] ( Fig. 1a ). Simultaneous time-lapse observation of Sec13-GFP and mRFP-Sed5 indicated an interesting behaviour of cis -Golgi cisternae ( Fig.1a ). cis -Golgi marked by mRFP-Sed5 showed repeated approach to the ERES and temporary association with it for a certain period of time (2–6 s). In contrast, the motion of trans -Golgi (Sec7-mRFP) looked random in relation to the ERES. They happened to pass by near the ERES, but no appreciable association was observed. Furthermore, we frequently observed a decrease in the fluorescence signal of Sec13-GFP, when cis -Golgi leaves the ERES after the association. 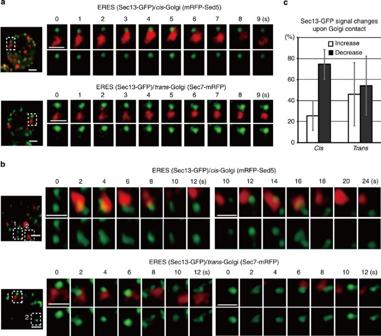Figure 1:cis-Golgi shows approach-and-contact actions towards the ERES. Wild-type cells expressing Sec13-GFP (COPII coat protein, green) with mRFP-Sed5 (cis-Golgi, red) and Sec7-mRFP (trans-Golgi, red) were observed with SCLIM. (a) Behaviours ofcis-Golgi (n=21 from 14 cells) andtrans-Golgi (n=48 from 28 cells). Representative two-dimensional (2D) images are shown on the left. Right panels show time-lapse images (one frame per second) of boxed areas. Scale bar, 1 μm. (b) Seven optical slices 0.1 μm apart around the centre of cells were taken at 0.15-s intervals. Three-dimensional (3D) images were reconstructed into movies (Supplementary Movies 1 and 2), of which representative views (boxed areas) are shown in the right panels. Scale bar, 1 μm. (c) Sec13-GFP signal changes on the contact ofcis-andtrans-Golgi are shown (cis-Golgi,n=113 from 13 cells;trans-Golgi,n=122 from 33 cells). Figure 1: cis- Golgi shows approach-and-contact actions towards the ERES. Wild-type cells expressing Sec13-GFP (COPII coat protein, green) with mRFP-Sed5 ( cis -Golgi, red) and Sec7-mRFP ( trans- Golgi, red) were observed with SCLIM. ( a ) Behaviours of cis- Golgi ( n =21 from 14 cells) and trans- Golgi ( n =48 from 28 cells). Representative two-dimensional (2D) images are shown on the left. Right panels show time-lapse images (one frame per second) of boxed areas. Scale bar, 1 μm. ( b ) Seven optical slices 0.1 μm apart around the centre of cells were taken at 0.15-s intervals. Three-dimensional (3D) images were reconstructed into movies ( Supplementary Movies 1 and 2 ), of which representative views (boxed areas) are shown in the right panels. Scale bar, 1 μm. ( c ) Sec13-GFP signal changes on the contact of cis- and trans- Golgi are shown ( cis -Golgi, n =113 from 13 cells; trans -Golgi, n =122 from 33 cells). Full size image SCLIM is based on the combination of high-speed spinning-disk confocal scanning, ultrahigh-sensitivity detection and data processing. The thickness of the confocal plane in the spinning-disk method is 1–2 μm. To confirm that the temporary association between cis -Golgi and the ERES was indeed their contact and that the decrease in the COPII coat signal was real, we performed 3D dual-colour time-lapse observation. Figure 1b shows an example of projections of such 3D movies. Here, clearer images indicate that cis -Golgi cisternae perform approach-and-contact actions (this behaviour can be likened to a ‘hug-and-kiss’) towards the ERES (note the merge of red and green signals) and then leave. Such intimate association was rarely observed between trans -Golgi and the ERES. As for the fluorescence signals of Sec13-GFP, Fig. 1b shows examples that they were significantly decreased. We made a statistical analysis for the changes of Sec13-GFP signals after the contact with Golgi cisternae ( Fig. 1c ). Because the fluorescence signals fluctuate, there were always random increase and decrease, but the case of cis -Golgi showed a clear bias towards the decrease as compared with trans -Golgi (see also Supplementary Movies 1 and 2 ). cis- Golgi is stuck at the ERES when secretion is compromised We next asked whether the ‘hug-and-kiss’ action of cis- Golgi to the ERES was affected when secretion was compromised. Glucose deprivation has been known to impair protein secretion in S. cerevisiae and cause slowing down of Golgi cisternal maturation and coalescence of the ERES [18] . 3D images of glucose-deprived cells showed that the proportion of cis- Golgi cisternae associated with the ERES increased (26±10% with glucose and 63±23% without glucose (mean±s.d. )), whereas trans- Golgi remained mostly separate from the ERES (7±8% with glucose and 4±8% without glucose) ( Fig. 2a,b ). 3D time-lapse images of mRFP-Sed5 and Sec13-GFP in glucose-deprived cells demonstrated that cis- Golgi cisternae were largely stuck at the ERES and the Sec13-GFP signal did not decrease ( Fig. 2c ). Persistent contact between cis- Golgi and the ERES was also observed in cells treated with cycloheximide to block protein synthesis ( Fig. 3 ). 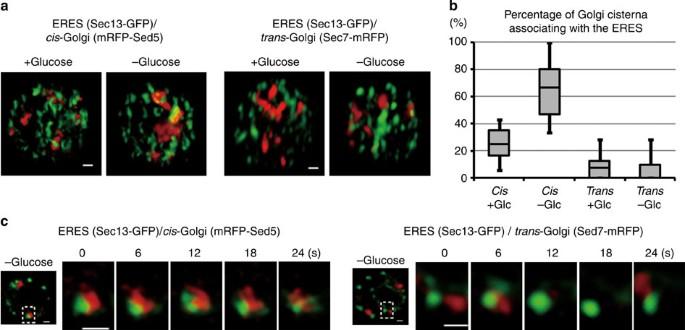Figure 2:cis-Golgi is stuck at the ERES when secretion is compromised. Wild-type cells expressing Sec13-GFP (COPII coat protein, green) and mRFP-Sed5 (cis-Golgi, red) or Sec7-mRFP (trans-Golgi, red) were grown to a mid-log phase. Culture was changed to a fresh medium with or without glucose (Glc). Image acquisition started 5 min after the medium change. (a) Representative 3D images of a whole cell. (b) The percentages ofcis-ortrans-Golgi associating with the ERES are shown in a box plot. The horizontal line in each box represents the median value of the distribution. The boundaries of a box represent the lower and upper quartile values. The whiskers extending vertically from the lower and upper portions of each box represent the extent of the rest of the data. (cis-Golgi,n=243 from 19 cells with glucose andn=222 from 35 cells without glucose;trans-Golgi,n=239 from 24 cells with glucose andn=209 from 31 cells without glucose). (c) Seven optical slices 0.1 μm apart around the centre of cells were taken at 0.15-s intervals. Representative 3D time-lapse images of an ERES andcis-Golgi ortrans-Golgi (boxed areas) in glucose-deprived cells are shown. Figure 2: cis- Golgi is stuck at the ERES when secretion is compromised. Wild-type cells expressing Sec13-GFP (COPII coat protein, green) and mRFP-Sed5 ( cis -Golgi, red) or Sec7-mRFP ( trans- Golgi, red) were grown to a mid-log phase. Culture was changed to a fresh medium with or without glucose (Glc). Image acquisition started 5 min after the medium change. ( a ) Representative 3D images of a whole cell. ( b ) The percentages of cis- or trans- Golgi associating with the ERES are shown in a box plot. The horizontal line in each box represents the median value of the distribution. The boundaries of a box represent the lower and upper quartile values. The whiskers extending vertically from the lower and upper portions of each box represent the extent of the rest of the data. ( cis -Golgi, n =243 from 19 cells with glucose and n =222 from 35 cells without glucose; trans -Golgi, n =239 from 24 cells with glucose and n =209 from 31 cells without glucose). ( c ) Seven optical slices 0.1 μm apart around the centre of cells were taken at 0.15-s intervals. Representative 3D time-lapse images of an ERES and cis- Golgi or trans- Golgi (boxed areas) in glucose-deprived cells are shown. 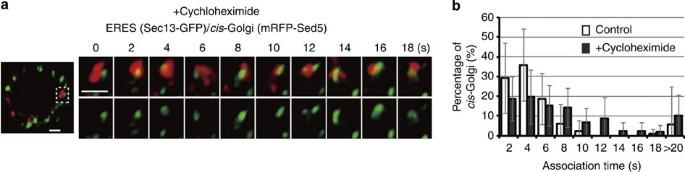Figure 3: Persistent contact betweencis-Golgi and the ERES in cells treated with cycloheximide. Wild-type cells expressing Sec13-GFP (COPII coat protein, green) and mRFP-Sed5 (cis-Golgi, red) were grown to a mid-log phase and then treated with 100 μg ml−1cycloheximide for 30 min. (a) Seven optical slices 0.1 μm apart around the centre of cells were taken at 0.15-s intervals. Representative 3D time-lapse images of an ERES andcis-Golgi (boxed areas) in glucose-deprived cells are shown. (b) Contact time between Sec13-GFP (COPII coat protein) and mRFP-Sed5 (cis-Golgi) in cells treated with or without cycloheximide (control,n=72 from 12 cells; with cycloheximide,n=155 from 12 cells). Full size image Figure 3: Persistent contact between cis- Golgi and the ERES in cells treated with cycloheximide. Wild-type cells expressing Sec13-GFP (COPII coat protein, green) and mRFP-Sed5 ( cis -Golgi, red) were grown to a mid-log phase and then treated with 100 μg ml −1 cycloheximide for 30 min. ( a ) Seven optical slices 0.1 μm apart around the centre of cells were taken at 0.15-s intervals. Representative 3D time-lapse images of an ERES and cis- Golgi (boxed areas) in glucose-deprived cells are shown. ( b ) Contact time between Sec13-GFP (COPII coat protein) and mRFP-Sed5 ( cis -Golgi) in cells treated with or without cycloheximide (control, n =72 from 12 cells; with cycloheximide, n =155 from 12 cells). Full size image cis- Golgi is stuck at the ERES in tether-impaired cells Biochemical studies have revealed that the directionality of traffic from the ER to the Golgi is controlled by the sequential interactions between COPII coats and tethering factors [19] , [20] . The tethering complex TRAPPI contains the activity as the guanine-nucleotide exchange factor for Ypt1 and binds to Sec23. TRAPPI activates Ypt1 thereby inducing binding between Ypt1 and its effector Uso1, a long coiled-coil tethering protein localizing on the Golgi membrane. Subsequently, the protein kinase Hrr25 (ref. 21 ) localizing on the Golgi phosphorylates Sec23/24 complex, which facilitates shedding of COPII coats. This suggests that COPII coats are not removed from the membrane until reaching the Golgi membrane. We examined the relationship between the ERES and cis -Golgi in the uso1-1 cells, which lack the Uso1 tethering function at the restrictive temperature (37 °C) [22] . As shown in Fig. 4 , under this condition, cis -Golgi stayed associated with the ERES (17±12% at 25 °C and 47±16% at 37 °C) ( Fig. 4a,b ) without invoking the decrease in Sec13-GFP signals ( Fig. 4c ). trans- Golgi was still freely moving in the cytoplasm (5±6% at 25 °C and 4±5% at 37 °C) ( Fig. 4c ). Taken together, these findings suggest that COPII coats are released only when normal functions of Uso1 and other transport machinery are fulfilled. 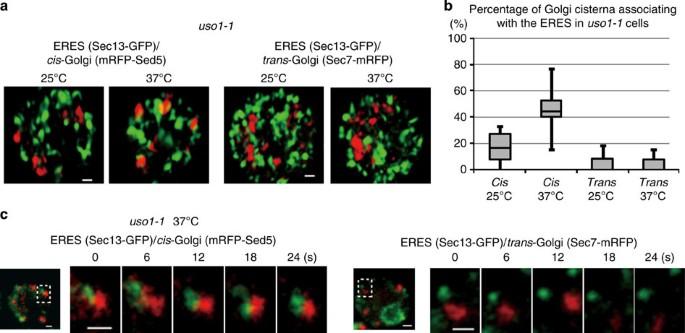Figure 4:cis-Golgi is stuck at the ERES when Uso1 function is impaired. uso1-1cells expressing Sec13-GFP (COPII coat protein, green) and mRFP-Sed5 (cis-Golgi, red) or Sec7-mRFP (trans-Golgi, red) were cultured at permissive (25 °C) or restrictive (37 °C) temperature for 30 min. (a) Representative 3D images of a whole cell are shown. (b) The percentages ofcis-ortrans-Golgi associating with the ERES are shown in a box plot. The horizontal line in each box represents the median value of the distribution. The boundaries of a box represent the lower and upper quartile values. The whiskers extending vertically from the lower and upper portions of each box represent the extent of the rest of the data (cis-Golgi,n=250 from 19 cells at 25 °C andn=209 from 18 cells at 37 °C;trans-Golgi,n=217 from 20 cells at 25 °C andn=141 from 15 cells at 37 °C). (c) Representative 2D time-lapse images of an ERES andcis-Golgi ortrans-Golgi (boxed areas) in cells at the restrictive temperature are shown. Scale bar, 1 μm (a,c). Figure 4: cis- Golgi is stuck at the ERES when Uso1 function is impaired. uso1-1 cells expressing Sec13-GFP (COPII coat protein, green) and mRFP-Sed5 ( cis -Golgi, red) or Sec7-mRFP ( trans- Golgi, red) were cultured at permissive (25 °C) or restrictive (37 °C) temperature for 30 min. ( a ) Representative 3D images of a whole cell are shown. ( b ) The percentages of cis- or trans- Golgi associating with the ERES are shown in a box plot. The horizontal line in each box represents the median value of the distribution. The boundaries of a box represent the lower and upper quartile values. The whiskers extending vertically from the lower and upper portions of each box represent the extent of the rest of the data ( cis -Golgi, n =250 from 19 cells at 25 °C and n =209 from 18 cells at 37 °C; trans -Golgi, n =217 from 20 cells at 25 °C and n =141 from 15 cells at 37 °C). ( c ) Representative 2D time-lapse images of an ERES and cis- Golgi or trans- Golgi (boxed areas) in cells at the restrictive temperature are shown. Scale bar, 1 μm ( a , c ). Full size image Cargo is transiently loaded into the ERES Our data imply an intriguing possibility that cis- Golgi captures cargo at the ERES via the hug-and-kiss action. Live cell visualization of cargo transport along the secretory pathway had been a big challenge, but we succeeded in setting up a system to do so. We chose a GFP-tagged cargo Axl2-GFP, a transmembrane protein targeted to the plasma membrane of the bud tip [23] , and expressed it under a heat-shock promoter ( SSA1 ) [24] in the temperature-sensitive sec31-1 mutant. The sec31-1 mutant is defective in the assembly of the Sec31 coat at the restrictive temperature (39 °C). At this temperature, new synthesis of Axl2-GFP was induced but the COPII budding was blocked. Thus, the cargo Axl2-GFP accumulated in the ER of these cells ( Fig. 5a , upper panel). On temperature shift-down to 25 °C, the cells were restored from the COPII-budding block and Axl2-GFP, whose new synthesis was repressed, started export from the ER and went on to the Golgi ( Fig. 5a , lower panel). Cargo loading into the ERES was observed in sec31-1 cells expressing heat-shock-induced Axl2-GFP and constitutive Sec13-mRFP ( Fig. 5b ). Two-dimensional time-lapse images showed that a small portion of cargo was loaded into the ERES on release from the COPII-budding block; the cargo signal then disappeared from the ERES coincidently with a decrease in the signal of Sec13-mRFP ( Fig. 5b,c ). 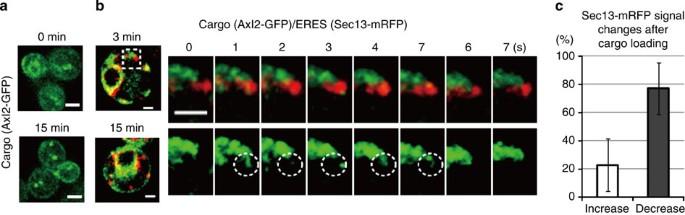Figure 5: Cargo is transiently loaded into the ERES. (a) When cultured at 39 °C for 30 min,sec31-1cells harbouring theAXL2-GFPgene under the control of the heat-shock promoter (SSA1) had induced synthesis of Axl2-GFP (0 min). COPII budding was blocked at 39 °C because of thesec31-1temperature-sensitive mutation. On temperature shift-down to 25 °C on the microscopic stage, cells were released from the COPII-budding block and Axl2-GFP began to be exported from the ER and went on to the Golgi apparatus (15 min). Scale bar, 2 μm. (b)sec31-1cells expressing heat-shock-inducible Axl2-GFP (cargo, green) and constitutive Sec13-mRFP (COPII coat, red) were released from the COPII-budding block and then imaged (left panels). Representative 2D time-lapse images of Axl2-GFP and an ERES (boxed areas) are shown in the upper right panels. Dotted circle indicates Axl2-GFP co-localizing with the ERES. The lower right panels are high-contrasted images to show the small amount of Axl2-GFP. Scale bar, 1 μm. (c) Sec13-mRFP signal changes after Axl2-GFP loading into the ERES (n=91 from 20 puncta of Sec13-mRFP in 12 cells). Figure 5: Cargo is transiently loaded into the ERES. ( a ) When cultured at 39 °C for 30 min, sec31-1 cells harbouring the AXL2-GFP gene under the control of the heat-shock promoter ( SSA1 ) had induced synthesis of Axl2-GFP (0 min). COPII budding was blocked at 39 °C because of the sec31-1 temperature-sensitive mutation. On temperature shift-down to 25 °C on the microscopic stage, cells were released from the COPII-budding block and Axl2-GFP began to be exported from the ER and went on to the Golgi apparatus (15 min). Scale bar, 2 μm. ( b ) sec31-1 cells expressing heat-shock-inducible Axl2-GFP (cargo, green) and constitutive Sec13-mRFP (COPII coat, red) were released from the COPII-budding block and then imaged (left panels). Representative 2D time-lapse images of Axl2-GFP and an ERES (boxed areas) are shown in the upper right panels. Dotted circle indicates Axl2-GFP co-localizing with the ERES. The lower right panels are high-contrasted images to show the small amount of Axl2-GFP. Scale bar, 1 μm. ( c ) Sec13-mRFP signal changes after Axl2-GFP loading into the ERES ( n =91 from 20 puncta of Sec13-mRFP in 12 cells). Full size image cis- Golgi captures cargo at the ERES To visualize the behaviour of cargo in relation to ERES-to-Golgi transport, we next examined sec31-1 cells that constitutively expressed Mnn9-mCherry, a subunit of Golgi mannosyltransferase complex that localizes mainly in cis- Golgi [25] tagged with mCherry [26] , and the heat-shock-inducible Axl2-GFP. After the temperature shift to 25 °C, Axl2-GFP was exported from the ER to the Mnn9-mCherry-labelled cis -Golgi ( Fig. 6a , left panels). 2D and 3D time-lapse images of Mnn9-mCherry and Axl2-GFP demonstrate that cis- Golgi began to associate with a particular region of the ER, most probably the ERES, and captured cargo. Then the cis- Golgi left the ER together with the cargo ( Fig. 6a,b , and Supplementary Movies 3–5 ). 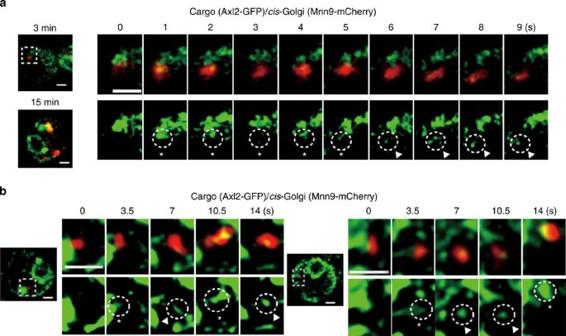Figure 6:cis-Golgi captures cargo at the ERES. sec31-1cells expressing heat-shock-inducible Axl2-GFP (cargo, green) and constitutive Mnn9-mCherry (cis-Golgi, red) were released from the COPII-budding block and then imaged. (a) Axl2-GFP is partly co-localized withcis-Golgi (left panels). Right panels show representative 2D time-lapse images of Axl2-GFP andcis-Golgi (boxed area). (b) 3D images were reconstructed from 15 optical slices 0.1 μm apart around the centre of cells taken at 0.2-s intervals (left panels). Right panels show representative 3D time-lapse images of Axl2-GFP andcis-Golgi (boxed areas). Dashed circles, Axl2-GFP contained incis-Golgi. Asterisks, Axl2-GFP captured bycis-Golgi. Arrowheads, Axl2-GFP leaving from the ER together withcis-Golgi. The lower panels are high-contrasted images to show the small amount of Axl2-GFP. Scale bar, 1 μm (a,b). Figure 6: cis- Golgi captures cargo at the ERES. sec31-1 cells expressing heat-shock-inducible Axl2-GFP (cargo, green) and constitutive Mnn9-mCherry ( cis- Golgi, red) were released from the COPII-budding block and then imaged. ( a ) Axl2-GFP is partly co-localized with cis -Golgi (left panels). Right panels show representative 2D time-lapse images of Axl2-GFP and cis -Golgi (boxed area). ( b ) 3D images were reconstructed from 15 optical slices 0.1 μm apart around the centre of cells taken at 0.2-s intervals (left panels). Right panels show representative 3D time-lapse images of Axl2-GFP and cis -Golgi (boxed areas). Dashed circles, Axl2-GFP contained in cis- Golgi. Asterisks, Axl2-GFP captured by cis- Golgi. Arrowheads, Axl2-GFP leaving from the ER together with cis- Golgi. The lower panels are high-contrasted images to show the small amount of Axl2-GFP. Scale bar, 1 μm ( a , b ). Full size image Our data have clearly demonstrated that yeast cis- Golgi contacts the ERES, by what we would call a hug-and-kiss action, and captures cargo during this contact (see Fig. 7 for our model). Our findings suggest that COPII vesicle do not necessarily have to be released into the cytosol. They can be captured by cis -Golgi before the release. This mechanism appears to be much safer than forming many free COPII vesicles in the cytosol and also explains why COPII vesicles are not easily found in electron micrographs of normally grown cells. Of course we do not rule out the possibility that free COPII vesicles are released and the cis -Golgi just immediately captures them. Previous examples of close association between the ERES and the Golgi have been known for invertebrates, plants and budding yeast P. pastoris , in which COPII vesicles are captured by the Golgi quickly after release [3] , [4] , [5] . Even with mammalian cells, an elaborate EM study previously showed that the ERES and the vesicular tubular cluster (ERGIC) are organized in a highly specialized zone and suggested that COPII vesicles were tethered as they formed [27] . The mechanism we are proposing ensures efficient and targeted ER-Golgi cargo transport even in the species like S. cerevisiae that does not have highly organized Golgi structures. 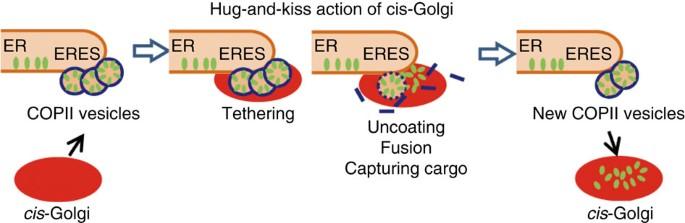Figure 7: A model of ER-Golgi cargo transport by a ‘hug-and-kiss’ action ofcis-Golgi. The ERES localizes on high-curvature ER domains such as on ER tubules or at the edge of ER sheets, and cargo protein (green) synthesized in the ER is loaded into the ERES.cis-Golgi (red large ellipse) performs an approach-and-contact (hug-and-kiss) action towards the ERES. During contact between COPII buds/vesicles andcis-Golgi, the COPII coat (blue line) cage collapses.cis-Golgi that received cargo then leaves the ERES. Figure 7: A model of ER-Golgi cargo transport by a ‘hug-and-kiss’ action of cis- Golgi. The ERES localizes on high-curvature ER domains such as on ER tubules or at the edge of ER sheets, and cargo protein (green) synthesized in the ER is loaded into the ERES. cis -Golgi (red large ellipse) performs an approach-and-contact (hug-and-kiss) action towards the ERES. During contact between COPII buds/vesicles and cis- Golgi, the COPII coat (blue line) cage collapses. cis -Golgi that received cargo then leaves the ERES. Full size image Secretory cargoes vary in size; therefore, some cargo proteins, such as procollagen fibres in mammalian cells, are too large to load into conventional COPII vesicles, and oversized vesicles have been postulated to generate to accommodate secretion of such large cargoes [28] , [29] . The oversized COPII vesicles may not have to be sealed and released if our proposed mechanism operates. A big question remains how the cis- Golgi finds the ERES. Actin and microtubule cytoskeletons probably do not play a role here, because cis- Golgi in S. cerevisiae moves independently of these cytoskeletons. Some matrix-like protein might stabilize the interaction between the ERES and the cis -Golgi. TFG protein of C. elegans and mammals is an interesting candidate [3] , [30] , but yeast does not seem to have its close homologue. Tethers such as the TRAPPI complex and Uso1 are intriguing players that could guide the cis -Golgi to the ERES, and if so the word ‘hug’ would be appropriate. The functions of these tethers in hug-and-kiss actions will of course be a target of our future studies. We previously demonstrated that yeast Golgi cisternae mature over time; the cis -Golgi changes its nature via medial-Golgi to trans- Golgi [7] , [31] . An interesting question would be whether the cis -Golgi approaching the ERES goes into the maturation phase immediately after contact. In the glucose deprivation experiment ( Fig. 3 ), a certain fraction of cis -Golgi was left unassociated with ERES, even though there are more ERES than cis -Golgi in number [8] . This might be because there are two populations of c is -Golgi, one for capture of cargo from the ERES (hug-and-kiss) and the other for carbohydrate modification (maturation). The former cis -Golgi could be regarded as similar to the mammalian ERGIC. Recent studies on plant Golgi support this view [4] , [32] . We have already made a substantial progress towards simultaneous multicolour observation at high-speed and super-high-resolution [9] and will fully utilize it to address these and other unresolved questions by live cell imaging. Yeast strains, plasmids and culture conditions Yeast cells were grown in MCD medium (0.67% yeast nitrogen base without amino acids (Difco Laboratories ), 0.5% casamino acids (Difco Laboratories ) and 2% glucose) with appropriate supplements. For live imaging, cells were grown to a mid-log phase at 25 °C. Strains expressing fluorescent protein-tagged Sec13, Mnn9 were constructed by a PCR-based method using pFA6a plasmids as a template, which is described in the yeast GFP database at the University of California, San Francisco [33] (primers 5′-TTTATGGAAGGAAAATCTTGAGGGTAAATGGGAACCCGCTGGTGAAGTTCATCAGCG GATCCCCGGGTTAATTAA-3′ and 5′-CTCATTTGCATTCTTTTTTCTTTTGAGATGTTTCATTTTAAATTCTTGATACTCTGAATT CGAGCTCGTTTAAAC-3′ for Sec13 and primers 5′-ATTTGGCTTACCAAACTATTTGGTTTATCACATAGAGGAAGAGAACCATCGGATCCCC GGGTTAATTAA-3′ and 5′-ATTATCTTTCAATAACGCTATAGCTTCTGTATGCTTTTTGCTCAGTTGCGAATTCGAGC TCGTTTAAAC-3′ for Mnn9). mRFP-Sed5 was expressed under the control of the TDH3 promoter on the low-copy plasmid pRS316 (ref. 34 ). Sec7-mRFP was expressed similarly except that the ADH1 promoter was used instead of the TDH3 promoter. Axl2-GFP was expressed under the control of a heat-shock promoter on the low-copy plasmid pRS316 or on the integrated plasmid pRS304. Fluorescence microscopy Cells were immobilized on glass slides using concanavalin A and imaged by SCLIM. SCLIM was developed by combining an Olympus model IX-71 inverted fluorescence microscope with a UPlanSApo × 100 NA 1.4 oil objective lens (Olympus, Japan), a high-speed and high-signal-to-noise-ratio spinning-disk confocal scanner (Yokogawa Electric, Japan), a custom-made spectroscopic unit, image intensifiers (Hamamatsu Photonics, Japan) equipped with a custom-made cooling system and two EM-CCD cameras (Hamamatsu Photonics, Japan) for green and red observation [9] . For raising space resolution, a magnification lens (4 or × 10) was put in the light path between the confocal scanner and the spectroscopic unit. For 3D images, we collected optical sections spaced 0.1 μm apart in stacks by oscillating the objective lens vertically with custom-made piezo actuator (Yokogawa Electric) relative to sample planes. Typically, 80 optical sections could span whole cells. For 3D time-lapse images, we took sequential 7 or 15 optical sections around the centre of a cell. Volocity software (Perkin Elmer, MA) was used to reconstruct and deconvolve 3D images via point-spread functions optimized for our spinning-disk confocal scanner. MetaMorph software (Molecular Devices, CA) was used for showing time-lapse images and for fluorescence signal change analysis. A thermo-controlled stage (Tokai Hit, Japan) was used to observe temperature-sensitive mutants. How to cite this article: Kurokawa, K. et al. Contact of cis- Golgi with ER exit sites executes cargo capture and delivery from the ER. Nat. Commun. 5:3653 doi: 10.1038/ncomms4653 (2014).